A troodontid dinosaur from the latest Cretaceous of India Troodontid dinosaurs share a close ancestry with birds and were distributed widely across Laurasia during the Cretaceous. Hundreds of occurrences of troodontid bones, and their highly distinctive teeth, are known from North America, Europe and Asia. Thus far, however, they remain unknown from Gondwanan landmasses. Here we report the discovery of a troodontid tooth from the uppermost Cretaceous Kallamedu Formation in the Cauvery Basin of South India. This is the first Gondwanan record for troodontids, extending their geographic range by nearly 10,000 km, and representing the first confirmed non-avian tetanuran dinosaur from the Indian subcontinent. This small-bodied maniraptoran dinosaur is an unexpected and distinctly ‘Laurasian’ component of an otherwise typical ‘Gondwanan’ tetrapod assemblage, including notosuchian crocodiles, abelisauroid dinosaurs and gondwanathere mammals. This discovery raises the question of whether troodontids dispersed to India from Laurasia in the Late Cretaceous, or whether a broader Gondwanan distribution of troodontids remains to be discovered. Theropod dinosaurs dominated terrestrial ecosystems, especially within predatory niches, for much of the Mesozoic, attaining a cosmopolitan distribution by the Early Jurassic. Within Theropoda, however, there are clear palaeogeographic divisions, especially among faunas from the Late Cretaceous (100.5–65.5 million years ago, or Megannum (hereafter, Ma)) [1] , [2] . For example, abelisauroids make a substantial contribution to theropod diversity in the Late Cretaceous of Gondwana, with abelisauroid occurrences in South America, Africa, Madagascar, India and Europe [3] . However, noasaurids, a clade of small-bodied abelisauroids, are not confidently known from Laurasia [4] . Instead, small-bodied Laurasian theropods of this age are exclusively maniraptorans, representing the ecologically diverse theropod clade that includes birds. Only a depauperate maniraptoran assemblage is known from the Cretaceous of Gondwana, comprising birds, alvarezsaurids and endemic unenlagiine dromaeosaurids [2] , [5] , and thus far lacking several groups, including the close avian relatives Troodontidae. The only specimen of a possible Gondwanan troodontid described to date, a manual ungual from the Cretaceous of Sudan [6] , likely represents a noasaurid abelisauroid instead [7] . Tetanurae, a large, globally distributed dinosaur group that includes Maniraptora and most Cretaceous theropod diversity is not yet known from Mesozoic deposits of the Indian subcontinent [8] . Although many Indian dinosaur remains discovered over the last two centuries were originally identified as coelurosaurian or ‘carnosaurian’ theropods (for example, in a study by Huene and Matley [9] ), these taxa have since been redescribed as abelisauroids, including some small-bodied noasaurids [3] , [10] and, in the case of a Late Triassic specimen [11] , as a basal saurischian [12] . Indeed, at present the earliest record of tetanurans in India is an Eocene bird [13] . Whether the Mesozoic absence in India of this large and common dinosaur clade is the result of historically limited sampling or represents a real palaeobiogeographic pattern has remained uncertain. Late Cretaceous vertebrate faunas of India hail almost entirely from infra- and intertrappean deposits in the Deccan volcanic province. These beds have yielded several theropod taxa, including Indosuchus , Indosaurus [14] , Rajasaurus [15] and Rahiolisaurus [16] , as well as the only confirmed Gondwanan eutherian mammals [17] , [18] , [19] , [20] , [21] . In contrast to the relatively rich record from infra- and intertrappean beds of Central India, comparatively few vertebrate fossils [22] , [23] have been described from the Cauvery Basin, comprising an extensive sequence of Early Cretaceous to Early Palaeocene fossiliferous sediments in Tamil Nadu, South India [24] ( Fig. 1 ). Since 2007, we have engaged in a comprehensive survey of the Cretaceous vertebrate fauna of the Cauvery Basin, which thus far has yielded hexanchid, lamniform, and hybodontiform sharks and ichthyosaurs from the marine deposits of the Cenomanian Karai Formation [25] , [26] and abelisauroid dinosaurs, Simosuchus- like notosuchian crocodyliforms and indeterminate ganoid fishes, anurans, crocodyliforms and turtles from the continental deposits of the Late Maastrichtian-aged (about 70.6–65.5 Ma) Kallamedu Formation [27] . Most of the terrestrial taxa occurring in the Kallamedu Formation are also previously known from the sedimentary beds of the Deccan volcanic province or from other Gondwanan continents, and the Simosuchus- like notosuchian indicates close faunal affinities with Madagascar in particular [27] . 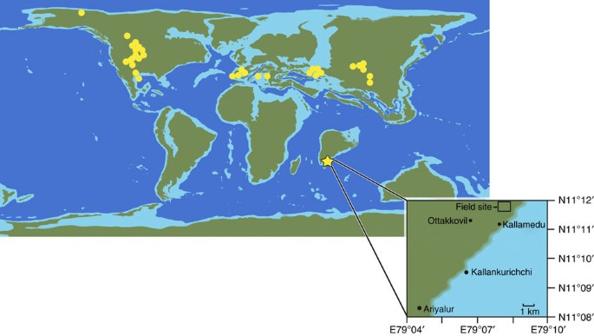Figure 1: Late Cretaceous distribution of Troodontidae. (a) Palaeogeographic reconstruction of the latest Cretaceous (∼65.5 Ma) showing previously known occurrences of Troodontidae (yellow circles) and location of the new specimen described here (yellow star). Occurrence data were downloaded from the Paleobiology Database on 30 November 2012 using the group name ‘Troodontidae’ and the following parameter: time interval, Late Cretaceous. Inset shows locality information for the Kallamedu Formation field site in the Cauvery Basin, Tamil Nadu, South India, projected on approximate palaeocoastline. Palaeogeographic map modified from reconstructions by Ron Blakey, NAU Geology (http://jan.ucc.nau.edu/∼rcb7/065Marect.jpg). Figure 1: Late Cretaceous distribution of Troodontidae. ( a ) Palaeogeographic reconstruction of the latest Cretaceous ( ∼ 65.5 Ma) showing previously known occurrences of Troodontidae (yellow circles) and location of the new specimen described here (yellow star). Occurrence data were downloaded from the Paleobiology Database on 30 November 2012 using the group name ‘Troodontidae’ and the following parameter: time interval, Late Cretaceous. Inset shows locality information for the Kallamedu Formation field site in the Cauvery Basin, Tamil Nadu, South India, projected on approximate palaeocoastline. Palaeogeographic map modified from reconstructions by Ron Blakey, NAU Geology ( http://jan.ucc.nau.edu/ ∼ rcb7/065Marect.jpg ). Full size image Here we describe an unusual dinosaurian tooth recovered by screenwashing at a microvertebrate site in the Kallamedu Formation that differs markedly from any previously known specimens from the Indian subcontinent or its palaeogeographic neighbours. This new specimen is identified as a troodontid dinosaur, representing the first record of Troodontidae in Gondwana and the first Mesozoic maniraptoran, and tetanuran, from India. This new discovery expands the Cretaceous geographic range of troodontids by nearly 10,000 km and further complicates understanding of the origin and affinities of India’s Cretaceous fauna. Geological setting The Cauvery Basin is a large northeast-southwest trending structure that formed during the Late Jurassic–Early Cretaceous rifting of India and Australia-Antarctica [28] . The sedimentary succession has been divided into three lithostratigraphic units: the Uttatur Group, the Trichinopoly Group and the Ariyalur Group, in ascending superpositional order. The focus of this study is on the youngest of these units, the Ariyalur Group, which is extensively exposed to the east and northeast of the town of Ariyalur. The dinosaurian tooth described here was recovered from screenwashing of 300 kg of sandy clays from the Kallamedu Formation, which forms the uppermost beds of the Ariyalur Group and has been assigned a Late Maastrichtian age based on planktonic foraminferans [29] , [30] . The Kallamedu Formation is exposed in a restricted area to the northeast of the small village of Kallamedu, ∼ 10 km north of Ariyalur ( Fig. 1 ), and consists of conspicuous red clays, friable sandstones and sandy clays, which have been interpreted as representing a fluvial, flood-plain environment in a coastal setting [31] . Before our current survey [27] , vertebrate fossil discoveries from the Kallamedu Formation were limited to fragmentary material of indeterminate sauropod and theropod dinosaurs [23] , [32] and well-preserved crania and postcrania of a bothremydid turtle [22] . Institutional abbreviations DUGF, Delhi University, Geology Department, Fossil Catalogue, Delhi, India. Systematic palaeontology Referred material One isolated tooth (DUGF/52). Formation and age Kallamedu Formation, Ariyalur Group, Late Maastrichtian age. Description DUGF/52 measures 2.8 mm in fore-aft basal length and 3.5 mm in height. It is lanceolate and labiolingually compressed, with a slight lingual inclination. It has a lenticular cross-section, with an anterior keel. The apex is recurved, with a convex mesial carina, in labial or lingual view ( Fig. 2a ). The distal carina is only weakly concave, appearing almost straight in labial or lingual view, and is inclined more steeply than the mesial carina. An apicobasally oriented buttress is apparent medially on the lingual surface, and the lingual surface is concave mesially and distally to this buttress ( Fig. 2c ). The labial surface of the tooth is convex mesiodistally. A mesiodistal constriction is observed at the base of the crown. 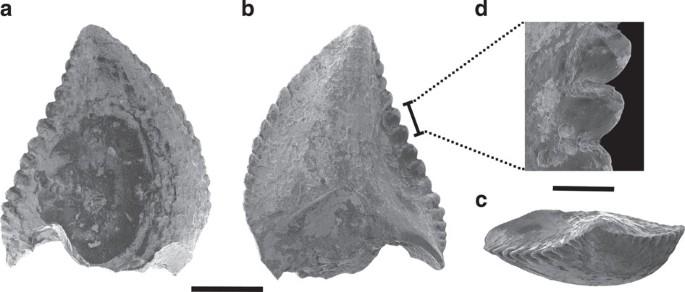Figure 2: New troodontid dinosaur from the latest Cretaceous of India. Troodontid tooth DUGF/52 in (a) labial, (b) lingual and (c) occlusal views, as well as a higher magnification view (d) of the distal denticles showing clear and well-formed interdenticle grooves despite abrasion (scale bar: 300 microns).a,bandcare shown at a uniform scale (with 1 mm scale bar). Images were obtained using a scanning electron microscope housed in the Department of Earth Sciences, University College London. Figure 2: New troodontid dinosaur from the latest Cretaceous of India. Troodontid tooth DUGF/52 in ( a ) labial, ( b ) lingual and ( c ) occlusal views, as well as a higher magnification view ( d ) of the distal denticles showing clear and well-formed interdenticle grooves despite abrasion (scale bar: 300 microns). a , b and c are shown at a uniform scale (with 1 mm scale bar). Images were obtained using a scanning electron microscope housed in the Department of Earth Sciences, University College London. Full size image The denticles are apically inclined, and relatively large, with a maximum apicobasal length of 0.25 mm at approximately midlength of both carinae. This length decreases towards the tooth apex and base. The denticles of the distal carina project further mesiodistally from the crown than do those of the mesial carina ( Fig. 2d ). Thus, the distal denticles appear larger in both lingual and labial views. The distal carina bears denticles along its entire height, to the basal constriction. However, the mesial carina seems to have terminated before reaching the base (although the situation is slightly obscured by damage to the base of the tooth, this morphology appears to be genuine). The denticles on the mesial carina have straight mesial borders and have a parallelogram-shaped outline in labial view due to their apical inclination (of approximately 45°). They are longer apicobasally than mesiodistally. The distal carina denticles have rounded distal margins and are longer mesiodistally than apicobasally. These denticles are perpendicular to the long axis of the crown at the base of the carina, but are slightly apically inclined midlength along the carina. Grooves are well-developed between adjacent denticles, reaching the base of the denticles on both carina, but do not extend onto the crown surface ( Fig. 2d ). DUGF/52 resembles the teeth of troodontids, a maniraptoran clade known only from North America and Eurasia, in the presence of a lingual buttress, presence of a basal constriction, the shape in labial view (which is most similar to the mesial maxillary and equivalent dentary teeth of troodontids [33] , [34] ), and the proportional size and apical inclination of the denticles. The proportional denticle size relative to the fore-aft basal length of the tooth is most similar to the troodontid Sinornithoides youngi [5] , [34] , a basal troodontid from China (although it differs in the presence of denticles on both carinae, they are absent on the mesial carina of S. youngi ). The distal denticles of DUGF/52 do not appear to be strongly hooked, unlike in some troodontids [35] , but these denticles are abraded and incomplete ( Fig. 2 ). Furthermore, this morphology is present only in some derived troodontids [34] , [36] . Isolated theropod teeth are notoriously difficult to assign to specific taxa, and a number of other dinosaurian, and reptilian, taxa bear some, but not all, of these features. However, the suite of characters described here are unknown in any other Cretaceous reptile clade and strongly support an assignment of this specimen to Troodontidae. For example, troodontid teeth show some resemblance to those of the extant squamate Iguana iguana [37] , but among Cretaceous squamates, Iguana -like (lanceolate, denticulate) teeth are only known in the boreoteiioid Kuwajimalla kagaensis [38] . However, the basal constriction of K . kagaensis is weak and occurs over a proportionally longer apicobasal distance, the crown lacks substantial apicodistal curvature, and the denticles of both carinae are of similar size and are more strongly inclined apically. Russell and Dong [39] noted similarity between some therizinosaur theropod teeth and those of troodontids. However, therizinosaurs also differ from DUGF/52 in lacking substantial apicodistal curvature and having mesial and distal denticles of similar size and stronger apical inclination [39] , [40] , [41] . Finally, although the teeth of some Late Triassic and Early Jurassic ornithischian and sauropodomorph dinosaurs had Iguana -like characters, some of which are shared with troodontids [37] , [42] , these taxa were extinct by the Cretaceous. Moreover, while superficially similar, the teeth of all of these older taxa differ from troodontids in possessing only weak apical recurvature and more strongly apically inclined denticles. Among theropod dinosaurs known from other Gondwanan continents, none compare favourably with DUGF/52. Abelisauroids, including small noasaurids such as those previously described from India and Madagascar [15] , [43] , [44] , [45] , could be considered the most likely possibility, but they are markedly different from DUGF/52 in dental morphology, most obviously in denticle size and crown height. The only other Gondwanan maniraptorans identified at present are dromaeosaurids, known mainly from Argentina [46] , as well as from India’s close Cretaceous neighbour Madagascar [47] , [48] . However, their teeth also bear much smaller denticles (or lose them entirely) and higher crowns, as well as lacking a constriction between the base and root, and thus are distinct from the specimen described here [46] . Unnamed maniraptorans from the Lower Cretaceous of Australia are known only from isolated postcrania [49] and so cannot be directly compared with DUGF/52. Enamel microstructure has recently been suggested as a phylogenetically informative character for some dinosaurian clades [50] . Unfortunately, theropods display a large amount of homoplasy in these characters, and troodontids in particular are highly variable. The lack of diagnostic enamel microstructure for this clade argues against destructive sampling of the sole known specimen of this first Gondowanan troodontid, and India’s first Mesozoic avetheropod, at present, but future discoveries may allow for further analysis along these lines. The identification of a troodontid dentary tooth represents an unusual and surprising extension of the palaeogeographic and temporal range of this predominantly Laurasian clade into the Late Cretaceous of India. This discovery demonstrates that the faunas of poorly sampled Gondwanan regions (for example, India, Madagascar or Australia) may deviate from the classic African and South American fauna that informs the most widely held hypotheses of Cretaceous terrestrial biogeography [1] . Indeed, new discoveries of Gondwanan, as well as Laurasian, dinosaurs have increasingly challenged the simple model of an endemic Gondwanan terrestrial vertebrate fauna throughout the Cretaceous [49] . The presence of troodontids also further confounds biogeographic reconstructions of Late Cretaceous India. Fossil discoveries have demonstrated that India’s fauna was dominated by the expected primarily or exclusively Gondwanan clades (for example, notosuchian crocodyliforms, gondwanathere mammals and abelisauroid dinosaurs [27] ) in the Late Cretaceous, but this simple biogeographic pattern has already been complicated by the presence of gobiatine frogs and possible anguimorph lizards [51] of Laurasian origin, and at least one other predominantly or even exclusively Laurasian clade, eutherian mammals, represented by Deccanolestes (although there is debate over an enigmatic therian mammal from the Late Cretaceous of Madagascar [52] , [53] ). Palaeogeographic reconstructions of Late Cretaceous India are also hotly contested. Some reconstructions suggest that India was connected to East Africa via the Oman-Kohistan-Dras Island Arc in the latest Cretaceous [54] , whereas another suggests that it remained connected to Antarctica into the Late Cretaceous [55] . Still another analysis differs in reconstructing India as being at its peak isolation in the latest Cretaceous, with only indirect connection to Africa by overwater dispersal via Madagascar, from ∼ 83.5 Ma (ref. 56 ). Connections to Laurasian continents are even more unlikely in that reconstruction, with India separated from any northern island arcs by an estimated 1,500 km of ocean. While these vast oceanic barriers may have prevented dispersal of large vertebrates between Gondwanan landmasses [57] , or directly between India and Laurasian continents in the latest Cretaceous, the presence of definitive eutherian mammals in the latest Cretaceous of India demonstrates that at least some small terrestrial vertebrates were likely dispersing between India, Africa and Europe, directly or indirectly, during the Late Cretaceous [17] , [20] , [21] . The presence of a troodontid dinosaur in the latest Cretaceous of India may thus be the outcome of a dispersal event from Laurasia to India, or indicate an undersampled Gondwanan distribution for Cretaceous troodontids, consistent with the recent discovery of non-dromaeosaurid maniraptorans in Early Cretaceous deposits of Australia [49] . As troodontids are known from the Middle Jurassic [58] , it is possible that the presence of troodontids in India is the result of vicariance or dispersal before India’s Late Cretaceous isolation. Although its explanation remains to be further tested, this unexpected new Indian discovery dramatically expands the known distribution of Troodontidae and suggests that further exploration of Gondwanan fossil localiities, particularly for small vertebrates, may dramatically alter current understanding of vertebrate biogeography and the evolution of major dinosaurian and other vertebrate clades. Surface prospecting and specimen recovery Surface prospecting was undertaken in a large exposure of the Kallamedu Formation ( Fig. 1 ) during expeditions in 2007, 2009 and 2010, which revealed a large concentration of highly fragmentary large bones that likely represent dinosaur taxa and have been previously identified as titanosaur sauropods [32] . In addition, microsites with concentrations of ganoid fish scales, turtle carapace fragments, and abelisaurid theropod and crocodilian teeth [27] were identified during surface prospecting. The specimen described here was recovered during screenwashing of material gathered from one such microsite. How to cite this article: Goswami, A. et al . A troodontid dinosaur from the latest Cretaceous of India. Nat. Commun. 4:1703 doi: 10.1038/ncomms2716 (2013).